Social amoeba farmers carry defensive symbionts to protect and privatize their crops Agricultural crops are investments that can be exploited by others. Farmer clones of the social amoeba Dictyostelium discoideum carry bacteria to seed out new food populations but they also carry other non-food bacteria such as Burkholderia spp. Here we demonstrate that these farmer-carried Burkholderia inhibit the growth of non-farmer D. discoideum clones that could exploit the farmers’ crops. Using supernatants, we show that inhibition is due to molecules secreted by Burkholderia . When farmer and non-farmer amoebae are mixed together at various frequencies and allowed to complete the social stage, the ability of non-farmers to produce spores falls off rapidly with an increase in the percentage of farmers and their defensive symbionts. Conversely, farmer spore production is unaffected by the frequency of non-farmers. Our results suggest that successful farming is a complex evolutionary adaptation because it requires additional strategies, such as recruiting third parties, to effectively defend and privatize crops. Social dilemmas, in which individual good conflicts with collective good [1] , are common in nature [2] , [3] . For example, Dictyostelium discoideum social amoebas divide asexually until their bacterial food source runs out and then they aggregate and cooperate to form a multicellular fruiting body [4] , [5] . About 20% of the cells die in the process of building a stalk that puts spores (the other 80% of cells) in a position to be dispersed to better areas. The dilemma arises because groups form by aggregation; hence, stalk production by one clone can be exploited by others, sometimes called cheaters, which produce little or no stalk. In this case, although cheating occurs [6] , [7] , it is greatly reduced by a variety of means, including kin recognition and other mechanisms that make many groups clonal [5] , [8] , [9] , [10] , [11] ; thus, stalk cell altruism can be favoured by kin selection. Some clones of D. discoideum face another social dilemma. Farmer clones carry potentially exploitable food bacteria through their dispersing spore stage to seed out after dispersal [12] . This behaviour is costly because farmers leave some uneaten bacteria behind, reducing the farmer’s ultimate reproductive spore production. However, carrying bacteria pays when the spores are dispersed to areas without good food bacteria. The ability of farmers to bring bacteria that previously allowed them to flourish at another site now allows them to capitalize on available nutrients and increase their reproductive spore production. Agriculture is very rare in non-humans [13] , [14] , [15] , [16] , [17] , perhaps because of the social dilemma inherent in investing in crops that can be exploited by others. In addition, farming by humans is the classic setting for the social dilemma called the tragedy of the commons; each farmer who adds a cow to a common pasturage gains the whole benefit, while imposing most of the costs on others, so the pasture becomes overgrazed, to the detriment of all [18] . An even more basic tragedy of the commons is glossed over in this account. If the cows themselves become commons and anyone can harvest their milk or meat, no farmers would invest in them. Non-human farmers, which include some ants, termites, ambrosia beetles, marine snails and damselfish [13] , [14] , [15] , [16] , [17] , must somehow solve this second dilemma without the benefit of anything like human institutions [19] that guarantee property rights or a just division of goods. D. discoideum farmers produce a valuable crop that could be eaten by a non-farming competitor clone who does not pay the costs of farming, so why is farming evolutionarily stable? Living in high-relatedness groups should help but multiple D. discoideum clones often co-occur in 0.2 gm soil samples [20] and sometimes even in single fruiting bodies [8] ; thus, exploitation remains an important concern. All farmers raised in the lab with the food bacterium Klebsiella pneumoniae will carry it while retaining one or more of a number of other species [12] . Some of these carried bacteria are not good food sources. As bacterial species produce a wide range of chemical products including antibiotics, virulence factors and bacteriocins [21] , [22] , [23] , these non-food bacteria could have pathogenic effects; however, this seems inconsistent with the observed ability of farmers to proliferate as well as non-farmers [12] . Alternatively, these bacteria might provide a benefit other than food, for example, defending against non-farmer D. discoideum clones to help privatize farmers’ crops. Here we show that these non-food bacteria also provide advantages to their host; they secrete molecules that promote the growth of their host but inhibit the growth of non-farming conspecifics of the host. Thus, D. discoideum farmers privatize their crops by carrying defensive symbionts directed at competitors. 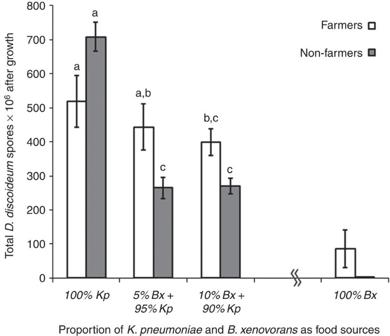Figure 1:Burkholderia xenovorans (Bx)is a poor food forD. discoideum. In 100%Bx,non-farmers are unable to produce any spores, whereas spore production for farmers is greatly reduced compared with 100%Klebsiella pneumoniae (Kp)control. However, small amounts ofBxharm non-farmer clones but not farmer clones. Non-farmers produce significantly fewer spores in 5%Bx+95%Kpand 10%Bx+90%Kpcompared with 100%Kpcontrol, whereas farmers have minimal change in spore production under the same conditions (mixed model analysis of variance: farmerF1,8=0.95,P=0.3588, treatmentF2,16=78.38,P<0.0001, farmer × treatmentF2,16=28.59,P<0.0001,n=10); Significant differences found between farmers and non-farmers are indicated by different letters, which reflect results of apost hocTukey’s honestly significantly different (HSD) test (this analysis excluded the 100%Bxtreatment that was not normally distributed and not directly relevant to the question of protecting a crop). Error bars equal s.e.m. Burkholderia xenovorans is inedible by D. discoideum To test this hypothesis, we used a set of 10 D. discoideum clones ( Table 1 ) consisting of 5 non-farmers and 5 farmers that carry bacteria B. xenovorans (>98% identity using a 481-bp PCR fragment of 16S ribosomal DNA for comparison), the most common non-food bacterium isolated from farmers. We separately cultured spores collected from these 10 D. discoideum clones, providing only B. xenovorans as a food source. Non-farmer D. discoideum clones were unable to grow in these pure cultures, with mortality so severe that spore production was zero ( Fig. 1 ). However, farmers were able to produce some spores in this treatment, although far fewer than when they are reared on a better food bacterium. It is not clear whether the farmer clones were eating B. xenovorans or whether they were feeding on carried K. pneumoniae that they had been grown on previously; however, it is clear that B. xenovorans carried by farmers is at best a very poor food source. Table 1 List of Dictyostelium discoideum clones used in each experimental assay. Full size table Figure 1: Burkholderia xenovorans (Bx) is a poor food for D. discoideum. In 100% Bx, non-farmers are unable to produce any spores, whereas spore production for farmers is greatly reduced compared with 100% Klebsiella pneumoniae (Kp) control. However, small amounts of Bx harm non-farmer clones but not farmer clones. Non-farmers produce significantly fewer spores in 5% Bx +95% Kp and 10% Bx +90% Kp compared with 100% Kp control, whereas farmers have minimal change in spore production under the same conditions (mixed model analysis of variance: farmer F 1,8 =0.95, P =0.3588, treatment F 2,16 =78.38, P <0.0001, farmer × treatment F 2,16 =28.59, P <0.0001, n =10); Significant differences found between farmers and non-farmers are indicated by different letters, which reflect results of a post hoc Tukey’s honestly significantly different (HSD) test (this analysis excluded the 100% Bx treatment that was not normally distributed and not directly relevant to the question of protecting a crop). Error bars equal s.e.m. Full size image B. xenovorans harm non-farmer but not farmer clones Normally, both B. xenovorans and a food bacterium like K. pneumoniae would be available to proliferating D. discoideum amoebae. Therefore, we also tested farmers and non-farmers on bacteria mixes with initial compositions dominated by K. pneumoniae but with 5 or 10% B. xenovorans mixed in. The smallest initial amount of B. xenovorans (5%) significantly reduced non-farmer spore production, yielding fewer than half as many spores as controls, whereas spore production for farmers was statistically unchanged ( Fig. 1 ). We found comparable results in the 10% B. xenovorans treatment, although with a slight reduction in farmer spores. This evidence is consistent with the hypothesis that B. xenovorans bacteria carried by farmers selectively harm their non-farmer D. discoideum competitors. B. xenovorans supernatants benefit farmers and harm non-farmers To test whether the reduction in non-farmer spore production is because of secreted biomolecules of B. xenovorans, we tested each of the same five farmer and five non-farmer clones against supernatants collected from each of the five farmers’ B. xenovorans isolates. For each of these 50 combinations, we plated out starved log-phase D. discoideum cells in four treatments. Treatment with supernatant was compared with control treatment with buffer only and this was crossed with treatments with or without the food bacterium K. pneumoniae (supernatant+food, buffer+food, no supernatant+food, buffer+no food). The treatments with bacterial food allowed us to assess bacterial supernatant effects on growing solitary vegetative cells (amoebae), measured as cell number after 3 h. Inhibition of non-farmers at this stage would most directly reduce their exploitation of a farmer’s crop. The treatments without bacteria induced starvation and fruiting to assess bacterial supernatant effects on spore production in the social stage. Killing non-farmers in this stage would lower the number of non-farmers co-dispersing with farmers, thereby reducing exploitation of farmers’ crops after dispersal. In both solitary (with food) and the social (without food) stages, we found that the supernatant caused harm to non-farmers and actually benefited farmers, relative to buffer controls ( Fig. 2 ). This pattern is evident at the individual level in each of the five supernatants ( Fig. 3 ) and is also evident at various solitary time points ( Fig. 4 ). This evidence verifies our hypothesis that secreted molecules from farmer-carried B. xenovorans bacteria specifically harm non-farmers and also suggests that farmers may have evolved some dependence on the secretions of their carried bacteria. 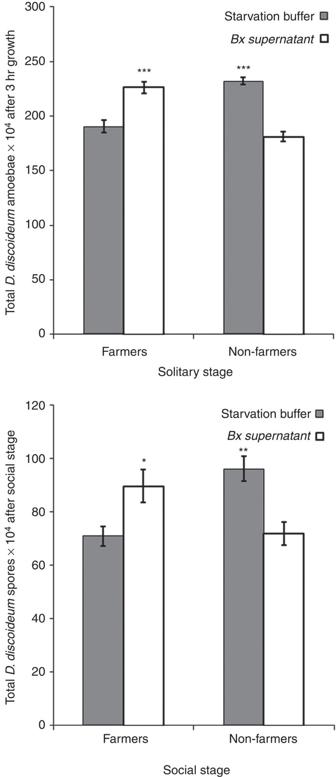Figure 2: Bacterial supernatants harm non-farmers and benefit farmers. Supernatants from farmer-associatedB. xenovoransisolates harm non-farmers and benefit farmers in the solitary, vegetative stage as well as the social stage. We tested 10 clones (5 farmers and 5 non-farmers) for amoebae and spore production inB. xenovorans. EachD. discoideumwas tested against all five supernatants, as well as five buffer controls and the averages were plotted. Non-farmers produce fewer amoebae and fewer spores in allB. xenovoranssupernatants compared with starvation buffer alone, whereas farmers consistently benefited from supernatants. Error bars equal s.e.m. *P<0.05, **P<0.005 and ***P<0.0005 (unequal-variance two-tailedt-tests, 7 df). Figure 2: Bacterial supernatants harm non-farmers and benefit farmers. Supernatants from farmer-associated B. xenovorans isolates harm non-farmers and benefit farmers in the solitary, vegetative stage as well as the social stage. We tested 10 clones (5 farmers and 5 non-farmers) for amoebae and spore production in B. xenovorans . Each D. discoideum was tested against all five supernatants, as well as five buffer controls and the averages were plotted. Non-farmers produce fewer amoebae and fewer spores in all B. xenovorans supernatants compared with starvation buffer alone, whereas farmers consistently benefited from supernatants. Error bars equal s.e.m. * P <0.05, ** P <0.005 and *** P <0.0005 (unequal-variance two-tailed t -tests, 7 df). 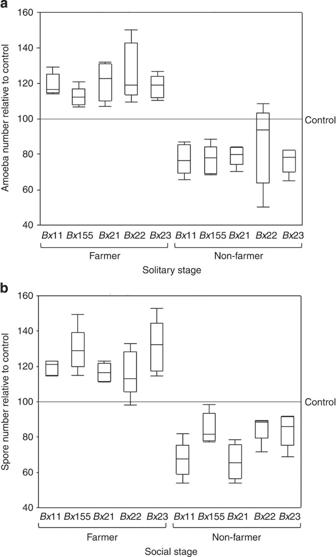Figure 3: Symbiont bacterial supernatants help farmers and harm non-farmers. Population pattern repeats at the individual level with all non-farmers producing significantly fewer amoebae and spores than farmers carryingB. xenovoransin all fiveB. xenovoranssupernatants. Farmers increase amoeba proliferation and spore production under the same conditions. We measured the change in amoeba proliferation (a) and spore production (b) in all fiveB. xenovoranssupernatants compared with either amoeba proliferation or spore production in a buffer control using 10 clones (5 farmers and 5 non-farmers) tested against 5B. xenovoranssupernatants individually prepared from 5 farmer-associated strains. Results are displayed as individual box plots. We used data from the 3-h logarithmic growth curve time point to display the solitary-stage box plots. Tails of box plots show minimum and maximum values. SeeFig. 4for all solitary-stage time points. Full size image Figure 3: Symbiont bacterial supernatants help farmers and harm non-farmers. Population pattern repeats at the individual level with all non-farmers producing significantly fewer amoebae and spores than farmers carrying B. xenovorans in all five B. xenovorans supernatants. Farmers increase amoeba proliferation and spore production under the same conditions. We measured the change in amoeba proliferation ( a ) and spore production ( b ) in all five B. xenovorans supernatants compared with either amoeba proliferation or spore production in a buffer control using 10 clones (5 farmers and 5 non-farmers) tested against 5 B. xenovorans supernatants individually prepared from 5 farmer-associated strains. Results are displayed as individual box plots. We used data from the 3-h logarithmic growth curve time point to display the solitary-stage box plots. Tails of box plots show minimum and maximum values. See Fig. 4 for all solitary-stage time points. 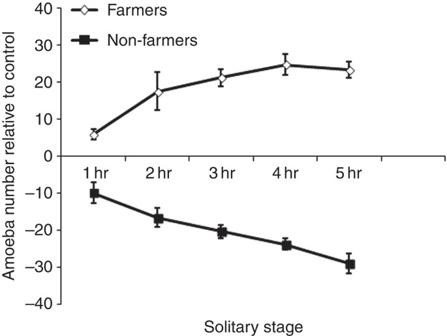Figure 4: Time course of vegetative amoeba proliferation inBurkholderia xenovorans (Bx)supernatants. We tested 10 clones (5 farmers and 5 non-farmers) for amoeba proliferation inBxsupernatants prepared from 5 individually isolated farmer-associated strains. We collected data for each clone with each supernatant every hour for 5 h. Harm to non-farmer amoebae increased as exposure time toBxsupernatants increased. Conversely, benefit to farmer amoebae increased with time under the same conditions. Error bars equal s.e.m. Full size image Figure 4: Time course of vegetative amoeba proliferation in Burkholderia xenovorans (Bx) supernatants. We tested 10 clones (5 farmers and 5 non-farmers) for amoeba proliferation in Bx supernatants prepared from 5 individually isolated farmer-associated strains. We collected data for each clone with each supernatant every hour for 5 h. Harm to non-farmer amoebae increased as exposure time to Bx supernatants increased. Conversely, benefit to farmer amoebae increased with time under the same conditions. Error bars equal s.e.m. Full size image Farmers are more competitive in mixtures with non-farmers Does this harming effect actually work when farmers and non-farmers are in direct competition? We performed ten pairwise sets of mixes of one farmer and one non-farmer at different frequencies ( Table 2 ). In addition to the farmer-associated bacteria B. xenovorans tested so far, we included farmers carrying bacteria identified as similar to B. phytofirmans , Burkholderia sp. CCGE1003 and Stenotrophomonas maltophilia ( Table 2 ). We paired each farmer with a non-farmer and for each pair tested five kinds of mixtures under starvation conditions, varying the percentages of the farmer and non-farmer in the mixtures: 100:0, 95:5, 50:50: 5:95, 0:100. After fruiting bodies matured, we determined the per capita spore return for both the farmer and non-farmer based on their original number of amoebae at the start of the experiment ( Fig. 5 ). We tested whether per capita spore production varies by farmer status and/or frequency by performing a two-way analysis of variance with replication. We found a significant effect of frequency, no significant effect of farmer status, but most interestingly, a strongly significant interaction between farmer/non-farmer status and frequency (mixed model analysis of variance: farmer F 1,18 =0.02, P =0.8886; frequency F 3,54 =14.13, P <0.0001; farmer × frequency F 3,54 =9.35, P <0.0001). Non-farmers alone produce more spores than farmers alone [12] . However, as the percentage of farmers increased, the per capita spore production of non-farmers was strongly reduced. In contrast, we found no change in the per capita spore production for farmers at the different mixture frequencies. Thus, increased frequency of the farmers and their carried bacteria seems to preferentially harm non-farmers. Table 2 List of D. discoideum farmer/non-farmer pairs and the host-associated potential defensive bacteria carried by the individual farmer. 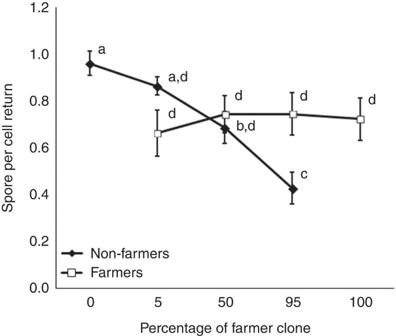Figure 5: Non-farmers lose competitively in mixes with farmers and their bacteria. Spore production decreases for non-farmers when mixed with farmers carrying their host-associated bacteria. We performed 10 sets of pairwise farmer:non-farmer mixes and found that non-farmers produce fewer spores per cell as the proportion of farmer in the mixture increases. Spore production for farmers is the same in all mixture conditions. Error bars equal s.e.m.;n=19. Significant differences found between spore outputs are designated by different letters as indicated by apost hocTukey’s HSD test. Full size table Figure 5: Non-farmers lose competitively in mixes with farmers and their bacteria. Spore production decreases for non-farmers when mixed with farmers carrying their host-associated bacteria. We performed 10 sets of pairwise farmer:non-farmer mixes and found that non-farmers produce fewer spores per cell as the proportion of farmer in the mixture increases. Spore production for farmers is the same in all mixture conditions. Error bars equal s.e.m. ; n =19. Significant differences found between spore outputs are designated by different letters as indicated by a post hoc Tukey’s HSD test. Full size image Linear regression of all non-farmer per capita spore production results on the percentage of the non-farmer at the different mixture frequencies with farmers explained 56.6% of the variance ( F 1,78 =101.852, P <0.001). It is worth asking whether this pattern is due to some subset of the experiments, perhaps because of differences in the bacterial species carried. All individual results for non-farmer spore production are consistent with the overall pattern ( Fig. 6 ). Nine out of 10 non-farmers decline significantly in spore production as the farmer frequency increases ( Table 3 ). Farmers carrying B. xenovorans , B. phytofirmans or S. maltophilia showed strong effects. The two smallest changes, one of them insignificant, were for the two farmers carrying Burkholderia sp. CCGE1003, suggesting that this species had a weaker effect. Nevertheless, these data support the hypothesis that B. xenovorans and other carried bacteria preferentially harm non-farmer D. discoideum in a dose-dependent manner. 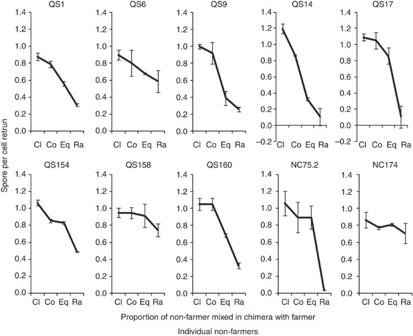Figure 6: Farmers dominate competitively over non-farmers at the individual level. Individual graphs of each non-farmer alone and mixed in chimera with a farmer at different frequencies. As farmer frequency increases in chimera with a non-farmer, 9 out of 10 non-farmers have significantly reduced spore production. We allowed 10 non-farmers to complete the social stage either alone (Cl=clonal or 100%) or mixed (Co=common or 95%, Eq=equal or 50%, or Ra rare or 5%) with farmers and determined the effect on the spores returned per initial cell of the non-farmer. Pairings and bacteria are shown inTable 2. Two independent replicas were performed; error bars equal s.e.m. Figure 6: Farmers dominate competitively over non-farmers at the individual level. Individual graphs of each non-farmer alone and mixed in chimera with a farmer at different frequencies. As farmer frequency increases in chimera with a non-farmer, 9 out of 10 non-farmers have significantly reduced spore production. We allowed 10 non-farmers to complete the social stage either alone (Cl=clonal or 100%) or mixed (Co=common or 95%, Eq=equal or 50%, or Ra rare or 5%) with farmers and determined the effect on the spores returned per initial cell of the non-farmer. Pairings and bacteria are shown in Table 2 . Two independent replicas were performed; error bars equal s.e.m. Full size image Table 3 Linear regression values for 10 individual non-farmers mixed at various frequencies with a paired farmer. Full size table The non-food bacteria carried by D. discoideum benefit their host while harming non-farmer clones. For the bacteria studied here, the chemistry is unknown but in another non-food symbiont, P. fluorescens , two small molecules (pyrollnitrin and chromene) have been identified as causing these effects [24] . How the bacteria can target some Dictyostelium clones without harming their host of the same species is a puzzle. A precedent exists with Caedibacter bacteria that kills competitors of their Paramoecium host clones [25] ; however, this raises two more questions. First, if the Dictyostelium symbionts can gain from targeting and harming non-farmers, why don’t they, like the Caedibacter symbionts, finish the job by evolved lethal effects? Second, why do only farmers carry defensive symbionts when non-farmers might also benefit from harming competitors? We suggest that these puzzles would be solved if the system arose not through the evolution of bacteria for specific targeting but primarily through the evolution of farmer resistance to sub-lethal effects. Farmers that carry food bacteria may inevitably pick up other bacteria. This side effect may initially be deleterious but if it is not lethal and if farming is advantageous enough to compensate for this disadvantage, the association may persist long enough for the farmer to evolve resistance to, and perhaps even dependence on, its new partner. Non-farmers would not incidentally pick up bacteria, and, without consistent exposure, would remain vulnerable at the original, non-lethal, level. Farming ants and beetles also carry bacteria used as defensive symbionts [26] , [27] , [28] . 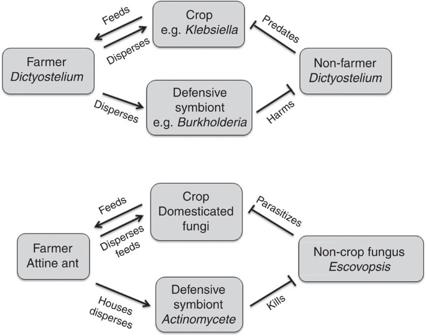Figure 7: Convergent evolution of symbiosis in ants and amoebae. D. discoideumand ant farmers reveal striking parallels in defence of their crops against exploitation. Solid arrows represent beneficial interactions such as food and dispersal; T-shaped bars represent harm. Figure 7 shows the striking parallels with the ant system. Crops provide food to the farmers. The farmers provide dispersal to the crops with the ants also practicing more complex cultivation by providing leaves for the fungus garden. Each farmer carries bacteria used for defence; whereas the ant’s bacteria attack a fungal parasite of the crop [29] , [30] , the bacteria carried by D. discoideum attack a predator of the crop that is a competitor of the farmer. For D. discoideum , this is the first evidence of some form of cultivation beyond dispersing and seeding their food crops. By carrying their defensive symbionts, they protect their crop bacteria from predators that offer no dispersal benefits and at the same time privatize the crop for their own use. Figure 7: Convergent evolution of symbiosis in ants and amoebae. D. discoideum and ant farmers reveal striking parallels in defence of their crops against exploitation. Solid arrows represent beneficial interactions such as food and dispersal; T-shaped bars represent harm. Full size image Culture conditions We grew all wild isolates from spores on SM/5 agar plates (2 g glucose, 2 g BactoPeptone (Oxoid), 2 g yeast extract (Oxoid), 0.2 g MgCl 2 , 1.9 g KH 2 PO 4 , 1 g K 2 HPO 4 and 15 g agar per litre) in association with bacteria K. pneumoniae at room temperature. Wild D. discoideum strains Our assays used a population of wild D. discoideum isolates collected at Mountain Lake Biological Station in Virginia (global positioning system coordinates: N 37° 21′, W 80° 31′) and Little Butt’s Gap, North Carolina. All clones with a QS designation were isolated from Mt. Lake Biological Station in Virginia and all clones with an NC designation were isolated from Little Butt’s Gap in North Carolina. Specific clones used for each assay are listed in Table 1 . Isolation of bacteria from wild D. discoideum farmer isolates We picked up the sorus contents of 6–12 random fruiting bodies grown on SM/5 plates in association with K. pneumoniae from each wild clone to be tested for farmer status using a filtered pipette tip. The sorus contents were spotted individually on SM/5 agar plates and assessed for bacterial growth after 2–5 days at room temperature. We collected bacteria from spots positive for growth using a sterile inoculating loop, resuspended the bacteria in 1 ml of starvation buffer (2.25 g KH 2 PO 4 and 0.67 g K 2 HPO 4 per litre H 2 O), vortexed and serially diluted in starvation buffer. We spotted the serial dilutions individually on SM/5 plates and collected individual colonies for species identification (for method see below in PCR amplification and sequence identification of novel bacteria). PCR amplification and sequence identification of novel bacteria We modified the procedures outlined in ‘Identifying Unknown Bacteria Using Biochemical and Molecular Methods’ found at http://www.nslc.wustl.edu/elgin/genomics/Bio3055/IdUnknBacteria06.pdf to prepare template DNA as stated below. From each novel bacterial isolate, we collected a small amount of stationary phase bacteria clonally grown on a nutrient agar plate and then resuspended the bacteria in 250 μl water (Sigma) in a 1.5-ml eppendorf tube. Next, we placed the tube of cells in a dry ice bath for 3 min. We transferred the tube to a 90 °C bath for 3 min. After repeating this cold/hot cycle for three times, we centrifuged the contents of the tube at 13,000 r.p.m. for 1 min. We collected the supernatant as the template DNA for PCR. The PCR amplification was done using a Gene Amp kit from Applied Biosystems (Roche). We used forward sequence 5′-CGG CCC AGA CTC CTA CGG GAG GCA GCA G-3′; and reverse sequence: 5′-GCG TGG ACT ACC AGG GTA TCT AAT CC-3′ as primers to amplify 481 bp of the 16S ribosomal RNA gene. We sequenced the PCR fragments generated (using the above procedure) at Lone Star Labs (Houston, TX) and used the NCBI web site as the search tool for sequences to identify bacteria to species. Log-growth amoebae preparation Three to five days after fruiting body formation, we individually collected spores from wild isolates in 1.5 ml eppendorf tubes containing about 400 μl of starvation buffer and determined spore density. To prepare log-growth amoebae, we plated 2 × 10 5 spores in 200 μl K. pneumoniae suspension in starvation buffer at an optical density (OD) of 1.5 A 600 on SM/5 plates. Using this plating regime, we previously determined that spore germination and amoeba log growth occurs at about 32–36 h after plating. When clones reached log-phase growth, we added 5 ml of ice-cold starvation buffer to the plate and collected the amoebae. Next, we centrifuged the collected amoebae/bacterial suspension at 1,500 g for 3 min to wash the amoebae clean of bacteria, and then we washed the pelleted amoebae in an excess volume of ice-cold starvation buffer three to four times depending on the amount of uneaten bacteria present. We determined the density of washed amoebae with dilution. D. discoideum spore production in B. xenovorans We tested spore production of five farmers and five non-farmers grown in 100% K. pneumoniae , 100% B. xenovorans , or a mixture of 5% B. xenovorans and 95% K. pneumoniae initial plating concentration or 10% B. xenovorans and 90% K. pneumoniae initial plating concentration. For this experiment, we used the B. xenovorans isolate from host farmer QS11. For the assay, we plated 2 × 10 5 spores of each clone in each of the four bacterial conditions onto SM/5 agar plates. All clones formed fruiting bodies by 3 days. We collected spores in a 15-ml conical tube by washing the plates with starvation buffer supplemented with 0.01% NP-40 alternative (about 10 ml for each clone) and measured the total volume collected for each. We vortexed each 15 ml conical tube briefly to evenly disperse the spores and determined the density by counting using a haemacytometer and a light microscope. Bacterial supernatant preparation We used five B. xenovorans isolates identified previously from five genetically different farmer strains as our test population of bacteria [12] . We prepared clonal isolates of each bacterial strain at the time of isolation from the farmer host and then stored them in 20% glycerol at −80 °C. For each experiment, we prepared the bacteria by starting from the frozen clonal isolate and then incubating at 21 °C until stationary phase was reached. For the experiment, we collected the stationary phase bacteria, placed the bacteria in a 30-ml conical tube containing starvation buffer, vortexed to obtain a homogeneous solution, determined the initial density using an Eppendorf BioPhotometer and then set the density to 1.5 A 600 by diluting with starvation buffer. To prepare the supernatant, we used a New Brunswick C1 Platform Shaker set at speed 25 to gently rotate the bacterial suspension for 1 h at 21 °C. Next, to isolate the bacterial supernatant from the bacteria, we centrifuged the bacterial suspension in an Eppendorf Centrifuge 5804 R at 12,000 g (13,000 r.p.m.) for 10 min at 4 °C. We decanted the supernatant to a fresh, sterile conical tube and placed the tube at 4 °C. Lastly, we filtered the supernatant through a 0.2-μm sterile syringe filter (Millipore) to remove any remaining live bacteria not removed by pelleting. We kept the prepared bacterial supernatant on ice until experimental set-up. At set-up, we prepared dilution of the supernatant in starvation buffer equivalent to the bacterial suspension set at OD 600 of 0.15. Supernatant experimental assay We collected log-growth amoebae from each of the 10 test clones as described above in ‘Culture conditions and mass plate preparation’. For the filter pad assay, we used 150 × 15 mm petriplates lined with two layers of WHATMAN NUMBER 3 , 125 mm circle filters (Schleicher & Schuell) soaked with either starvation buffer for the control or bacterial supernatant (see preparation above in ‘Bacterial supernatant preparation’) laid with a grid of equidistant 13 mm square AABP 04700 (Millipore, Bedford, MA) black filter squares. To test social stage spore production, we spotted the filters individually with 1.25 × 10 6 amoebae in starvation buffer and made duplicate samples for each clone for each experiment. We allowed the clones to hatch, grow and develop under direct light to limit potential movement of slugs before final culmination to fruiting bodies. Development was complete for all clones after about 24 h. We allowed the spores to mature in the fruiting bodies for an additional 24–48 h before collection. At that point, we collected each filter by placing the filter in a 1.5-ml conical eppendorf tube containing 1 ml starvation buffer+0.1% NP-40 alternative. We vortexed each eppendorf tube briefly to evenly disperse the spores and counted as above without dilution to determine density. We calculated spore number for experimental treatments as a percent change compared with control based on spore number recovered from starvation buffer control samples. To test amoeba proliferation in the solitary stage, we used the same basic set-up used above: We spotted filters individually and in duplicate with 5 × 10 5 log-growth amoebae in a K. pneumoniae /starvation buffer suspension set at an O.D. of 6.0 A 600 for each test clone. We collected filters every hour for 5 h after plating to determine the optimum time window for log growth versus exposure to the test bacterial supernatant ( Fig. 4 ). We collected each filter in 1 ml of starvation buffer and calculated the amoeba number for the experimental treatment as we did for the spore number above. Competition assay Using a population of 19 clones (10 non-farmers and 9 farmers), we competed each farmer against 1 unique non-farmer giving 10 pairwise mixes with 2 independent replicas performed for each pair. We paired one farmer with two different non-farmer clones. We prepared log-growth amoebae as above in ‘Culture conditions and mass plate preparation’. We labelled one clone of each pair fluorescently with Cell Tracker Green CMFDA (Invitrogen) to differentiate the clones in chimeras. Cell tracker in dimethylsulphoxide was added at a concentration of 6.67 μM to the clone being labelled and allowed time to be taken up by the cells. Then cells were washed free of unincorporated dye in starvation buffer during centrifugation. Unlabelled lines had an equal amount of dimethylsulphoxide without cell tracker added under the same conditions. We diluted all lines to a concentration of 5 × 10 7 cells ml −1 in ice-cold starvation buffer for the assay. We mixed D. discoideum clones labelled to unlabelled at the following non-farmer: farmer proportions: 5:95, 50:50 and 95:5. In addition, we plated both clones at 100% as controls for spore per cell productions. To assess for any labelling effects, we also plated the labelled line at 100%, as well as 50:50 labelled against unlabelled of the same clone and we saw no effects of labelling. We pipetted 25 μl of the control cells or mixes onto 0.8 μm pore size nitrocellulose filters (Millipore) placed individually on starving agar plates (0.36 gm Na 2 HPO 4 , 1.98 gm KH 2 PO 4 and 15 gm agar per 1 l H 2 O). After 3–5 days, we collected the filters and placed them in a 1.5-ml eppendorf tube containing 1 ml starving buffer+0.1% NP-40 alternative. After briefly vortexing the eppendorf tube, we measured the proportions of unlabelled and labelled cells and the number of cells per microlitre using an Accuri C6 flow cytometer. Data analyses For the Dictyostelium versus bacteria assay, the supernatant assays and the competition assay, we analysed our data using standard analysis of variance methodology with fixed effects (farmer and non-farmer) and a random effect (clone) with all possible interactions for all experimental assays. s.e. and F -statistics were KR-corrected [31] . The data analysis was generated using SAS software, Version 9–2 of the SAS System for Windows, Copyright 2002–2003, SAS Institute Inc. The regression analysis was analysed using SPSS Statistics 20, Release Version 20.0.0 (SPSS, Inc., 2011, Chicago, IL, http://www.spss.com ), with dependent variable as spore production and frequency as constant in the overall regression. In the individual regressions, frequency and clone were constant. The supernatant assays were additionally analysed using pairs between two groups (starvation buffer and B. xenovorans supernatant) for each clone using Student’s t -test. How to cite this article: Brock, D. A. et al . Social amoeba farmers carry defensive symbionts to protect and privatize their crops. Nat. Commun. 4:2385 doi: 10.1038/ncomms3385 (2013).